Modulating the frequency and bias of stochastic switching to control phenotypic variation Mechanisms that control cell-to-cell variation in gene expression (‘phenotypic variation’) can determine a population’s growth rate, robustness, adaptability and capacity for complex behaviours. Here we describe a general strategy (termed FABMOS) for tuning the phenotypic variation and mean expression of cell populations by modulating the frequency and bias of stochastic transitions between ‘OFF’ and ‘ON’ expression states of a genetic switch. We validated the strategy experimentally using a synthetic fim switch in Escherichia coli . Modulating the frequency of switching can generate a bimodal (low frequency) or a unimodal (high frequency) population distribution with the same mean expression. Modulating the bias as well as the frequency of switching can generate a spectrum of bimodal and unimodal distributions with the same mean expression. This remarkable control over phenotypic variation, which cannot be easily achieved with standard gene regulatory mechanisms, has many potential applications for synthetic biology, engineered microbial ecosystems and experimental evolution. The amount of phenotypic variation (also known as gene expression noise) in a cell population can determine fitness by affecting growth rate, robustness and adaptation [1] , [2] , [3] , [4] . Increased phenotypic variation resulting from the differentiation of cells into distinct phenotypes can enhance adaptation and growth in fluctuating environments and increase the robustness of the population to environmental stress [5] , [6] , [7] , [8] , [9] , [10] . Furthermore, when different phenotypes perform specialized tasks and there is cooperation between them, this can lead to complex behaviours and highly organized communities [11] , [12] , [13] . Decreased phenotypic variation, where every cell is as close as possible to an optimal level of gene expression that maximizes fitness (and consequently lower or higher expression has a fitness cost), is usually advantageous in constant environments [14] , [15] . Given the importance of the amount of phenotypic variation in bacterial populations for their fitness and their capacity for complex behaviours, being able to control it is potentially very useful in synthetic biology particularly for directed evolution. However, there are currently no systems that allow flexible and independent control of phenotypic variation. The most common strategies for regulating bacterial gene expression, which vary transcription factor binding and the ribosome binding sequence [16] , [17] , are designed to tune mean expression rather than phenotypic variation. These strategies produce a fixed relationship between mean expression and the amount of phenotypic variation [18] , [19] , [20] with high mean expression associated with low phenotypic variation and low mean expression associated with high phenotypic variation. With these regulatory systems it is not easy to achieve low mean expression with low phenotypic variation and high mean expression with high phenotypic variation. Gene expression can also be altered by reconfiguring the regulatory network (for example, altering the path length in transcriptional cascades) that can modify the relationship between mean expression and phenotypic variation; however, this approach to regulating phenotypic variation is too inflexible for many applications and is usually not tunable [21] , [22] , [23] . We propose a general strategy for tuning phenotypic variation termed ‘FABMOS’ (frequency and bias modulation of switching). FABMOS involves regulating stochastic transitions between distinct OFF and ON expression states of a genetic switch ( Fig. 1a ). In this system, one input modulates the frequency of transitions between the expression states (that is, k ON and k OFF vary but their ratio is constant and the second input modulates the bias of the transitions (that is, the ratio of k ON to k OFF varies). The frequency determines whether the phenotypic distribution is bimodal (low frequency) or unimodal (high frequency) (dark and light green lines respectively, Fig. 1b ). The unimodal distribution occurs at high transition frequencies because cells do not have sufficiently long periods with and without protein production in the ON and OFF states to create distinct expression levels. If the transition frequency is very high, transcription initiation in the ON state will be disrupted causing a decrease in the mean of the unimodal distribution (orange line, Fig. 1b ). The bias in the transition to the ON and OFF expression states will also affect the steady state bimodal and unimodal distributions (compare purple and light green lines, Fig. 1b ). In theory, FABMOS provides more control over phenotypic variation than transcription factor regulation alone because it allows the frequency of transcriptional bursts to be controlled as well as their duration [18] , [19] , [24] . 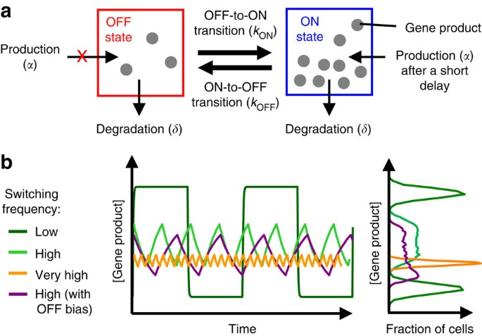Figure 1: General model of frequency and bias modulation of switching (FABMOS). (a) A two-state switch with random transitions and different expression levels for each state due to production of a gene product only occurring in the ON state. A general description of FABMOS is also described inSupplementary Note 1. (b) Representation of a time series showing the amount of gene product with switching between the OFF and ON states occurring at different frequencies (not to scale) and a fixed bias (that is,kONandkOFFvary but their ratio is constant) (left). The effect of the different frequencies on a population distribution with stochastic fluctuation in the amount of gene product is also shown (right). Figure 1: General model of frequency and bias modulation of switching (FABMOS). ( a ) A two-state switch with random transitions and different expression levels for each state due to production of a gene product only occurring in the ON state. A general description of FABMOS is also described in Supplementary Note 1 . ( b ) Representation of a time series showing the amount of gene product with switching between the OFF and ON states occurring at different frequencies (not to scale) and a fixed bias (that is, k ON and k OFF vary but their ratio is constant) (left). The effect of the different frequencies on a population distribution with stochastic fluctuation in the amount of gene product is also shown (right). Full size image In this study, FABMOS is evaluated as a strategy for controlling phenotypic variation and mean expression using the fim genetic switch (‘ fimS ’). The first part of the study shows using theoretical models and experiments that increasing the frequency of switching converts a bimodal distribution into a unimodal distribution, and that further increases in the frequency cause a graded decrease in the mean of the unimodal distribution. The second part shows that varying the bias as well as the frequency of switching between the ON and OFF states can generate a continuous spectrum of bimodal and unimodal phenotypic distributions with the same mean expression. Together, the findings demonstrate that FABMOS enables fine-tuning of phenotypic variation and mean expression in bacterial populations. Modulating the switching frequency A model of the fim genetic switch in Escherichia coli was created to directly examine the properties and behaviour of the FABMOS strategy in a realistic scenario ( Fig. 2a ). The advantages of modelling the fim system over a generic FABMOS system are that the assumptions can be minimized by incorporating experimental data, and the predictions can be tested experimentally (note: a general description of FABMOS is also provided in Supplementary Note 1 ). The fim switch has been used in synthetic circuits to prevent ‘leaky’ target gene expression [25] , generate multiple discrete states with other recombinase systems [26] and control chemotaxis [27] . 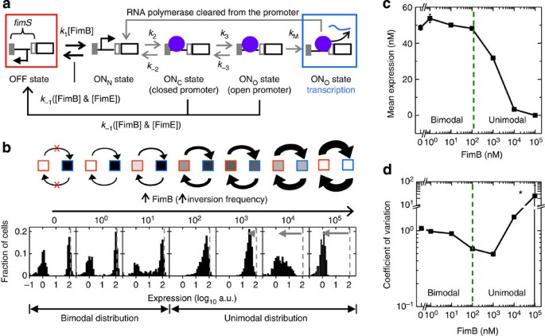Figure 2: Model offimswitch (fimS). (a) Diagram showing the regulation offimSby FimB and FimE and the steps required for transcription in the ON orientation (see main text). Purple circle represents RNA polymerase. (b) Histograms showing the simulated phenotypic distribution with increasing FimB concentration in a system without FimE (and with the initial fraction of ON cells being the steady state fraction of ON cells). The values above each histogram indicate the FimB concentration (a.u.). Grey arrows indicate the decrease in the median expression of the unimodal distribution from its maximum, which occurs at low concentrations of FimB (grey dash line). The schematic above each histogram shows the frequency of transition (increasing line thickness indicates increasing frequency), and the intensity of the grey shading in the red and blue squares indicates the relative level of gene expression in the OFF and ON orientations, respectively. Each histogram is generated from 400 simulated cells. (c,d) The mean expression and coefficient of variation (CV) for the phenotypic distributions shown inbat each FimB concentration. The green dash line indicates the approximate boundary between the bimodal and unimodal distributions. Error bars are the s.e.m. of duplicate simulations of 400 cells at each FimB concentration (totaln=14). *Error is large at the highest FimB concentration because CV values are being divided by very small mean expression values. SeeSupplementary Fig. 2for the mean expression and CV for a simulation where the initial inoculate has either all ON or all OFF cells to approximate the inoculation of a culture from an ON or OFF colony. Figure 2: Model of fim switch ( fimS ). ( a ) Diagram showing the regulation of fimS by FimB and FimE and the steps required for transcription in the ON orientation (see main text). Purple circle represents RNA polymerase. ( b ) Histograms showing the simulated phenotypic distribution with increasing FimB concentration in a system without FimE (and with the initial fraction of ON cells being the steady state fraction of ON cells). The values above each histogram indicate the FimB concentration (a.u.). Grey arrows indicate the decrease in the median expression of the unimodal distribution from its maximum, which occurs at low concentrations of FimB (grey dash line). The schematic above each histogram shows the frequency of transition (increasing line thickness indicates increasing frequency), and the intensity of the grey shading in the red and blue squares indicates the relative level of gene expression in the OFF and ON orientations, respectively. Each histogram is generated from 400 simulated cells. ( c , d ) The mean expression and coefficient of variation (CV) for the phenotypic distributions shown in b at each FimB concentration. The green dash line indicates the approximate boundary between the bimodal and unimodal distributions. Error bars are the s.e.m. of duplicate simulations of 400 cells at each FimB concentration (total n =14). *Error is large at the highest FimB concentration because CV values are being divided by very small mean expression values. See Supplementary Fig. 2 for the mean expression and CV for a simulation where the initial inoculate has either all ON or all OFF cells to approximate the inoculation of a culture from an ON or OFF colony. Full size image The fim system regulates the fimAICDFGH operon [28] encoding the FimA, FimI, FimC, FimD, FimF, FimG and FimH proteins that are either part of [29] or required for the synthesis [30] of type-1 fimbriae. The system is composed of a switch region ( fimS ) containing a promoter flanked by two inverted repeat sequences (IRL and IRR), which can be in an OFF or ON orientation. In the OFF orientation, the promoter is on the opposite DNA strand to the genes in the operon. The orientation of fimS is controlled by the FimB and FimE recombinases. FimB reportedly switches fimS in both directions at approximately equal rates (10 −2 –10 −3 cells·generation −1 ) in the absence of FimE [31] , [32] , [33] and thus, FimB controls the frequency of the transitions. FimE only inverts fimS from ON to OFF and thus it affects the bias . Note: reported feedback mechanisms between the fimE transcription and the fimS orientation are absent in the experimental system [34] because fimE is located on a plasmid away from fimS . In the ON orientation, transcription at the fim promoter is assumed to be a multistep process [35] , [36] and thus, there is a delay before it occurs after OFF-to-ON inversion ( Fig. 2a ). The first step is the conversion of the naked promoter (ON N state) to the ‘closed’ promoter (ON C state) by the binding of RNA polymerase. The second step is the formation of the open complex (ON O state). The third step is the transition to transcription elongation, which may occur after many abortive attempts, whereby RNA polymerase moves from the promoter and converts the ON O state to the ON N state. If fimS switches to the OFF orientation before these events are completed, then this transcription event will be aborted; if it does not, then transcription elongation will occur and additional transcription events may follow while the switch remains in the ON orientation. The maximum transcription rate of a constitutive promoter generates an mRNA approximately every 4 s (ref. 18 ; note: most promoters are not constitutively transcribed and therefore the period between transcription initiation events will be much greater than 4 s), which likely provides more than enough time for FimB or FimE to bind to the inversion sequences and disrupt transcription initiation or elongation. FimB and FimE will decrease mean expression if they affect any transcription event in the ON orientation, it does not have to be the first transcription event after fimS inverts to the ON orientation. Stochastic simulations of the model were performed to assess the effect of increasing the frequency of OFF-to-ON and ON-to-OFF transitions (that is, increasing FimB; see Methods). The simulations showed a bimodal distribution at low transition frequencies and then, as the frequency increases, the OFF and ON expression states merge into a unimodal distribution with an intermediate expression level that is approximately half the maximum expression (note: the distribution appears closer to the ON expression state on a logarithmic scale; Fig. 2b,c ). As mentioned above, the unimodal distribution occurs because cells are not in the OFF and ON orientations for sufficiently long periods for their expression levels to become distinct. Once the unimodal distribution arises, further increasing the frequency of the transitions causes a graded decrease in mean expression because cells have insufficient duration in the ON orientation to complete transcription. This graded decrease in expression does not occur if ( Supplementary Fig. 1 ): (i) FimB only regulates transitions in one direction (from OFF to ON); (ii) ON-to-OFF inversion only occurs when the promoter is in the ON N state (that is, bound RNA polymerase prevents inversion); and/or (iii) there is no delay in transcription because it is a single-step process. To evaluate how altering the fraction of OFF and ON orientation cells affects the phenotypic distributions, we calculated the coefficient of variation (CV) and the mean expression at different FimB concentrations. The CV is a simple metric for measuring the normalized amount of variation in the population. The CV is calculated by dividing the s.d. by the mean and it does not require any assumptions about the phenotypic distribution or fitting of any function. The latter is important because it is difficult to accurately deconvolve the OFF and ON expression states when their distributions overlap. In addition, the CV is a single metric that is sensitive to changes in the number and fraction of each expression state and the mean and variation of these states. As expected, we found that increasing the switching frequency by increasing FimB, so the two expression states become more similar, decreased the CV (that is, decreased phenotypic variation; Fig. 2b,d ). Further increases in switching caused the unimodal expression to decrease and this was accompanied by an increase in CV because mean expression falls at a faster rate than the variation in gene expression (as measured by the s.d.). These results are consistent with the patterns observed in the previous simulations and in simulations of cultures derived from OFF and ON colonies ( Supplementary Fig. 2 ). We constructed an experimental system based on the fim system to test the predicted effects of varying the frequency of transitions on the phenotypic distributions ( Fig. 3a ; Supplementary Fig. 3 ). The experimental system has the gfp gene at the position of fimA in the operon so that fimS in the ON orientation causes green fluorescent protein (GFP) production, which can be measured in single cells by flow cytometry. A similar system has been reported elsewhere [37] . We used GFP without a degradation tag to shorten its lifetime because even with the moderate strength AAV degradation tag [38] , the fluorescence was too low to distinguish between the OFF and ON states ( Supplementary Fig. 4 ). Chromosomal copies of fimB and fimE were deleted and their coding sequences were cloned under the control of inducible promoters (PLlacO-1 and PLtetO-1) with a ribosome binding sequence (st7) [39] on a medium copy plasmid [16] . PLlacO-1 and PLtetO-1 are regulated by the free concentration of LacI repressor and TetR repressor produced by a co-transformed plasmid. The amount of LacI and TetR repression is altered by adding different concentrations of isopropyl-β-D-thiogalactopyranoside (IPTG) and anhydrotetracycline (aTc), respectively, to the media. Due to the potency of ‘leaky’ FimE expression, fimE was not on the plasmid in experiments where we sought to vary only the frequency of transitions. The relative FimB and FimE levels at different IPTG and aTc concentrations were determined by placing gfp with the st7 RBS directly under the PLlacO-1 and PLtetO-1 promoters ( Supplementary Fig. 5 ). 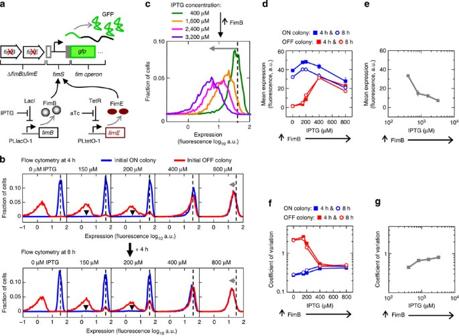Figure 3: Varying FimB expression in thefimexperimental system. (a) Schematic of the generalfimexperimental system. (b) Representative histograms of GFP expression in thefimsystem without FimE (HL4366) at 4 and 8 h after the addition of different IPTG concentrations (0, 150, 200, 400 and 800 μM). Cultures were inoculated with cells from OFF and ON colonies (red and blue lines, respectively). The experiment was performed in triplicate. Arrowheads highlight the small number of OFF cells in cultures derived from an ON colony. Note: in the far right panels, the distributions from the OFF and ON colonies overlay one another indicating a steady state distribution has been achieved. The dash line indicates the maximum expression level of the ON expression state and the grey arrow shows the decrease in average expression due to an increased frequency of switching at higher IPTG concentrations (and thus higher FimB concentrations). (c) Representative histograms of thefimsystem without FimE (HL4366) at high IPTG concentrations (400, 1,600, 2,400 and 3,200 μM). The experiment was performed in duplicate and cultures derived from ON and OFF colonies had the same histograms. (d,e) The mean expression for the experimental data corresponding tob(d) andc(e). Error bars are the s.e.m. of triplicate (totaln=60) and duplicate (totaln=8) measurements ford,e, respectively. (f,g) The coefficient of variation (CV) for the experimental data corresponding tob(f) andc(g). Error bars are the s.e.m. of triplicate (totaln=60) and duplicate (totaln=8) measurements forf,g, respectively. Figure 3: Varying FimB expression in the fim experimental system. ( a ) Schematic of the general fim experimental system. ( b ) Representative histograms of GFP expression in the fim system without FimE (HL4366) at 4 and 8 h after the addition of different IPTG concentrations (0, 150, 200, 400 and 800 μM). Cultures were inoculated with cells from OFF and ON colonies (red and blue lines, respectively). The experiment was performed in triplicate. Arrowheads highlight the small number of OFF cells in cultures derived from an ON colony. Note: in the far right panels, the distributions from the OFF and ON colonies overlay one another indicating a steady state distribution has been achieved. The dash line indicates the maximum expression level of the ON expression state and the grey arrow shows the decrease in average expression due to an increased frequency of switching at higher IPTG concentrations (and thus higher FimB concentrations). ( c ) Representative histograms of the fim system without FimE (HL4366) at high IPTG concentrations (400, 1,600, 2,400 and 3,200 μM). The experiment was performed in duplicate and cultures derived from ON and OFF colonies had the same histograms. ( d , e ) The mean expression for the experimental data corresponding to b ( d ) and c ( e ). Error bars are the s.e.m. of triplicate (total n =60) and duplicate (total n =8) measurements for d , e , respectively. ( f , g ) The coefficient of variation (CV) for the experimental data corresponding to b ( f ) and c ( g ). Error bars are the s.e.m. of triplicate (total n =60) and duplicate (total n =8) measurements for f , g , respectively. Full size image In the initial experiments, we induced different levels of FimB in exponentially growing cell cultures derived from OFF and ON orientation colonies and measured gene expression in single cells at 4 and 8 h after induction ( Fig. 3b ). At low FimB concentrations (up to ~200 μM IPTG) with low switching frequencies, we observed a bimodal distribution. At high FimB induction (~400 μM IPTG or greater) with high switching frequencies, we observed a unimodal distribution that shifted to lower mean expression levels as the FimB expression increased ( Fig. 3c–e ). Increasing the switching frequency also caused the CV in cultures derived from OFF colonies to decrease due to the two expression states converging (note: this was not apparent in cultures derived from ON colonies because there were too few OFF cells; Fig. 3f ). Further increasing the switching frequency caused the CV to increase as the mean expression decreased in the unimodal distribution ( Figs 2d and 3g ). The experimentally observed changes in the mean expression and CV with increasing FimB are very similar to that seen in the simulations ( Fig. 2c,d ; Supplementary Fig. 2 ). In summary, the mean expression and phenotypic variation in the experiments follow the general pattern associated with increasing frequency of switching predicted by the model. The decrease in mean expression with increasing FimB expression was not due to an indirect physiological effect. This was demonstrated by showing that high FimB concentrations have no effect on the expression of a gene encoding a red fluorescent protein (mCherry) under a constitutive promoter (HL6041; Supplementary Fig. 6 ) and no measurable effect on cell growth ( Supplementary Fig. 7 ). A fixed ratio of OFF and ON cells in unimodal distributions According to the model, the graded decrease in the unimodal distribution observed in the experiments is due to an increase in the frequency of transitions and not due to a change in the bias; this was confirmed by the following three methods. Our first method turned off FimB induction in unimodal distributions to ‘lock’ cells into their current fimS orientation. We then allowed cells time to grow and remove or accumulate proteins so the two expression states could become distinct, thereby enabling the fraction of cells in each state to be quantified. The experiment was performed at four IPTG concentrations (300, 400, 1,600 and 3,200 μM) that generate unimodal distributions with different mean expression levels. FimB induction was turned off by inoculating cells from media with IPTG into media without IPTG and growing them for 2 h. We found the same bimodal distribution occurred in all the samples despite their different prior levels of FimB induction (pink distribution, Fig. 4a ). The fractions of ON cells at 300, 400, 1,600 and 3,200 μM IPTG were similar: 75.3±1.1, 78.0±0.3, 76.9±0.5 and 78.9±0.1%, respectively. 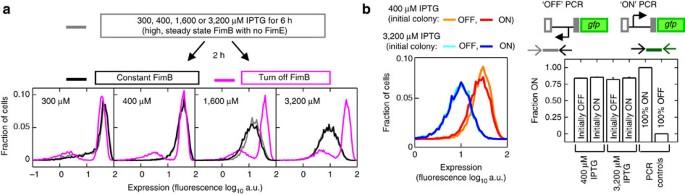Figure 4: The unimodal distributions are composed of a fixed ratio of both OFF and ON orientation cells. (a) Histograms of cells (HL4366) with different levels of FimB induction (grey line), which is then either turned off (magenta line) or maintained (black line). (b) Representative histograms for cells grown at 400 and 3,200 μM IPTG for 6 h. Cultures derived from OFF and ON expression colonies (HL4366) converged to the same distributions indicating they have reached steady state. The bar graph to the right shows the fraction of ON orientation cells in each distribution as determined by quantitative PCR. The scheme above the graph illustrates the relative positioning of the oligonucleotides used in separate reactions to amplifyfimSin the OFF and ON orientations (not to scale). The PCR controls werefimSPCR products in the OFF and ON orientations confirmed by DNA sequencing. Error bars are the s.e.m. of triplicate measurements for each column (totaln=12), except for the PCR controls which were duplicate measurements (totaln=4). Figure 4: The unimodal distributions are composed of a fixed ratio of both OFF and ON orientation cells. ( a ) Histograms of cells (HL4366) with different levels of FimB induction (grey line), which is then either turned off (magenta line) or maintained (black line). ( b ) Representative histograms for cells grown at 400 and 3,200 μM IPTG for 6 h. Cultures derived from OFF and ON expression colonies (HL4366) converged to the same distributions indicating they have reached steady state. The bar graph to the right shows the fraction of ON orientation cells in each distribution as determined by quantitative PCR. The scheme above the graph illustrates the relative positioning of the oligonucleotides used in separate reactions to amplify fimS in the OFF and ON orientations (not to scale). The PCR controls were fimS PCR products in the OFF and ON orientations confirmed by DNA sequencing. Error bars are the s.e.m. of triplicate measurements for each column (total n =12), except for the PCR controls which were duplicate measurements (total n =4). Full size image The second method measured the fimS orientation by quantitative PCR in two different unimodal distributions (400 and 3,200 μM IPTG) derived from OFF and ON colonies ( Fig. 4b ). The percentage of ON orientation cells was calculated from the relative amounts of product generated by PCRs that were specific for fimS in the ON and OFF orientations (see Methods). We found that the fraction of ON orientation cells at 400 and 3,200 μM IPTG was the same in cultures derived from ON colonies (85.3±0.6 and 84.2±1.3%, respectively) and OFF colonies (84.1±3.2 and 82.0±2.5%, respectively). The third method measured the inversion rates in bimodal distributions at low levels of FimB ( Fig. 3b ) to calculate the steady state fraction of ON orientation cells. The OFF-to-ON inversion rate was determined from the relative increase in the fraction of ON orientation cells in populations derived from OFF colonies at 4 and 8 h (there are negligible inversions in the reverse direction because the initial fraction of ON orientation cells is small; Fig. 3b ). Similarly, the ON-to-OFF inversion rate was obtained from the relative increase in the fraction of OFF orientation cells in populations derived from ON colonies (black arrowheads, Fig. 3b ). At 150 and 200 μM IPTG, the OFF-to-ON inversion rates were 24.7±4.1 × 10 −5 and 53.7±13.7 × 10 −5 min −1 , respectively, and the ON-to-OFF inversion rates were 4.5±2.9 × 10 −5 and 11.3±3.1 × 10 −5 min −1 , respectively. The ratio of OFF-to-ON and ON-to-OFF inversion is approximately the same at the two levels of FimB induction (4.8 and 5.5, respectively) despite a twofold difference in their rates. From these ratios, the predicted steady state fraction of ON orientation cells was determined to be 82.8 and 84.6% (that is, 4.8/(1+4.8) and 5.5/(1+5.5)). Previous studies found little-to-no bias in FimB inversion [31] , [32] , [33] . One explanation for the difference is that when we replaced both fimB and fimE genes with Kan R , the distal 230 bp of fimE was left intact to minimize effects that the sequence replacement might have on inversion of the neighbouring fimS (HL4366, Fig. 5a ). In contrast, other studies inactivated fimE with an IS 1 insertion sequence [31] , [33] and the exact sequence changes were not reported. It is possible that the latter method deleted flanking sequences that influence fimS inversion bias. We evaluated this possibility by creating two deletion strains; one strain has deleted all fimE up to its stop codon (HL6174) and the second strain has deleted all fimE plus the sequence between fimE and IRL (which is the 5′ boundary of fimS ; HL6189; Fig. 5a ). We found that the deletion of fimE up to its stop codon caused a small but significant decrease in the average fraction of ON orientation cells at 400 μM IPTG from 76.6±0.4% in our original strain to 63.5±3.5% (measured by the first method above; Fig. 5b ). The deletion of fimE plus the sequence between the end of fimE and the IRL sequence caused an even greater decrease in the average fraction of ON orientation cells at 400 μM IPTG from 76.6±0.7% in our original strain to 0.04±0.02% ( Fig. 5c ). Therefore, replacement of sequences flanking fimS can affect the switching bias. 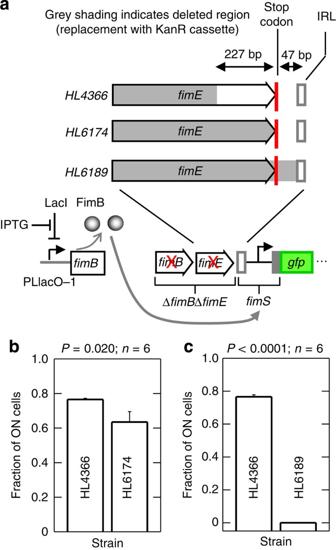Figure 5: The effect of deleting sequences that flankfimSon switching bias. (a) Schematic showing the different regions deleted and the experimental system. (b,c) Fraction of cells in the ON state at 400 μM IPTG after 8 h. Error bars are the s.e.m. of triplicate measurements (for each panel, totaln=6).Pvalues were calculated using a two-tailedt-test. HL4366 in panelsb,care separate experiments. Figure 5: The effect of deleting sequences that flank fimS on switching bias. ( a ) Schematic showing the different regions deleted and the experimental system. ( b , c ) Fraction of cells in the ON state at 400 μM IPTG after 8 h. Error bars are the s.e.m. of triplicate measurements (for each panel, total n =6). P values were calculated using a two-tailed t -test. HL4366 in panels b , c are separate experiments. Full size image A second explanation for the difference in the average fraction of ON orientation cells between our study and previous studies is methodological differences. We measured inversion rates in single cells in liquid culture using a GFP reporter, while previous studies determined the fraction of ON cells using the lacZ reporter assay (which requires cells to be plated on prewarmed solid agar with Xgal [33] ), colony morphology with immunofluorescence [32] or radiolabelling of DNA fragments extracted from single colonies [31] . We compared the fraction of ON orientation cells measured by flow cytometry (described above) and plating cells onto prewarmed solid agar. To do this, cells were first cultured in liquid Luria-Bertani (LB) media with 1 mM IPTG for 4 h to induce switching and then inoculated into LB media without IPTG for 2 h to turn-off FimB and ‘lock’ them into one orientation. The cultures were then taken to flow cytometry or plated (note: there were triplicate replicates of the culture). The latter was performed in duplicate for each culture and the plates were visualized by low-magnification fluorescent microscopy (× 4 objective) to count the fraction of single colonies with the ON and OFF expression states (note: only colonies with >90% of one expression state were counted). We found no significant difference in the fraction of ON orientation cells measured by the two methods (72.2±0.4% for flow cytometry and 69.6±3.8% for plating; two-tailed t -test: n =6, t -value=0.69, P =0.53). This result favours the first explanation for the difference in bias for the ON orientation between our study and others. In summary, FimB has a bias for OFF-to-ON inversions leading to a greater average fraction of ON orientation cells, which we show by the first (77.3±0.9%), second (83.9±0.8%) and third (83.7±1.3%) methods. Furthermore, the bias for the ON orientation does not change with the FimB concentration, it is the same in bimodal (at steady state) and unimodal distributions, and it does not impact the general behaviour of the FABMOS system (shown in simulations below). Modulating both the switching frequency and bias We next varied the bias as well as the frequency of transitions in our simulations. That is, there are two variable inputs: (i) FimB, which varies the switching frequency with a fixed bias; and (ii) FimE, which varies the bias by altering the transition rate from ON to OFF. FimB and FimE are assumed to have additive effects on ON-to-OFF inversion. The model includes the observed fivefold bias of FimB for OFF-to-ON inversion and assumes all cells are initially in the OFF orientation because cultures in the corresponding experiments were inoculated with cells from OFF colonies (see below). The simulations showed that at a fixed FimB concentration, increasing the FimE concentration increases the fractions of cells in the OFF expression state as expected ( Fig. 6a ). We further found that at a fixed FimE concentration, increasing the FimB concentration generated ‘loops’ when the CV is plotted as a function of the mean ( Fig. 6b ). This is a very different relationship to that of inducible promoters (for example, PLlacO-1), where the CV generally decreases with increased mean expression ( Supplementary Fig. 8 ) [19] . The loops start with no FimB and all the cells in the OFF orientation; therefore, there is minimal phenotypic diversity in the population (that is, a low CV) and low mean expression. As the FimB concentration increases, OFF-to-ON inversion can occur resulting in two expression states, which increases the CV and the mean. Further increasing FimB causes the transition frequency to increase, which decreases the difference in the expression states resulting in convergence to a unimodal distribution; this consequently decreases the CV and causes a net increase in mean expression for the population. Additional increases in FimB push the transition frequency to such a high level that the period for transcription initiation is truncated, leading to a reduction in mean expression and an increase in CV. 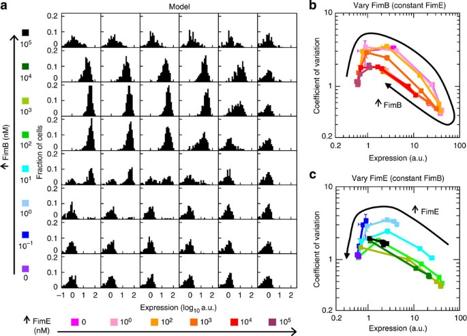Figure 6: Simulated effects of FimB and FimE on the phenotypic distribution. (a) Histograms generated by stochastic simulations showing the effect of increasing FimB concentration (bottom to top) and increasing FimE concentration (left to right). The relative concentrations (a.u.) of FimB and FimE are shown along the axes. (b) The coefficient of variation (CV) plotted as a function of mean expression for thefimsystem with increasing FimB concentrations and fixed FimE concentrations (equivalent to moving up the columns ina). Error bars are the s.e.m. of duplicate simulations of 400 cells for each combination of FimB and FimE concentrations (totaln=96). Data colours indicate the FimE concentrations ina. The solid lines are a guide for the eye. The arrow indicates the change in CV and mean expression with increasing FimB. (c) The CV plotted as a function of mean expression for thefimsystem with increasing FimE expression and fixed FimB concentrations (equivalent to moving left to right along the rows ina). Error bars are the s.e.m. of duplicate simulations of 400 cells for each combination of FimB and FimE concentrations (totaln=96). Data colours indicate the FimB concentrations ina. Solid lines guide the eye to a pattern observed at intermediate FimB concentrations that occurs experimentally (Fig. 7c). The arrow indicates the change in CV and mean expression with increasing FimE. Figure 6: Simulated effects of FimB and FimE on the phenotypic distribution. ( a ) Histograms generated by stochastic simulations showing the effect of increasing FimB concentration (bottom to top) and increasing FimE concentration (left to right). The relative concentrations (a.u.) of FimB and FimE are shown along the axes. ( b ) The coefficient of variation (CV) plotted as a function of mean expression for the fim system with increasing FimB concentrations and fixed FimE concentrations (equivalent to moving up the columns in a ). Error bars are the s.e.m. of duplicate simulations of 400 cells for each combination of FimB and FimE concentrations (total n =96). Data colours indicate the FimE concentrations in a . The solid lines are a guide for the eye. The arrow indicates the change in CV and mean expression with increasing FimB. ( c ) The CV plotted as a function of mean expression for the fim system with increasing FimE expression and fixed FimB concentrations (equivalent to moving left to right along the rows in a ). Error bars are the s.e.m. of duplicate simulations of 400 cells for each combination of FimB and FimE concentrations (total n =96). Data colours indicate the FimB concentrations in a . Solid lines guide the eye to a pattern observed at intermediate FimB concentrations that occurs experimentally ( Fig. 7c ). The arrow indicates the change in CV and mean expression with increasing FimE. Full size image FimE increases the fraction of cells in the OFF orientation at any given FimB concentration, which has the effect of decreasing both the CV and decreasing mean expression (that is, it ‘shrinks’ the loop; Fig. 6b ). When the FimE concentration is varied and the FimB concentration is constant, a ‘swirl’ pattern occurs ( Fig. 6c ). Altering both the FimB and the FimE concentrations (that is, altering both the frequency and the bias of switching) can generate many (that is, more than two) different distributions and CV values with the same mean expression level and conversely many different mean expression levels for a given CV value ( Fig. 6b,c ). We experimentally tested the predicted effects of varying the bias as well as the frequency of switching. The experiments were performed by taking cultures of cells derived from OFF colonies and adding different amounts of IPTG and aTc to the media to induce different FimB and FimE concentrations, respectively ( Fig. 7a ). At low FimB concentrations, we found that increasing FimE increased the fraction of cells in the OFF expression state (third row from bottom, Fig. 7a ). At high FimB concentrations, we found that increasing FimE shifted the unimodal distribution to a lower mean (third row from top, Fig. 7a ). These observations are consistent with the known role of FimE in increasing ON-to-OFF inversion of fimS . 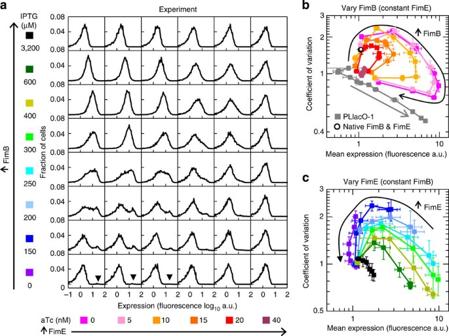Figure 7: The regulation offimSby FimB and FimE. (a) A 6 × 8 ‘phase plane’ of representative histograms for thefimSsystem at different combinations of FimB and FimE expression. The phase space was measured in quintuplicate (HL4234). Panels from left to right show increasing FimE induction and panels from bottom to top show increasing FimB induction. Arrowheads highlight the small subpopulation of cells with the ON expression state. (b) The coefficient of variation (CV) as a function of mean expression with varying FimB and a fixed amount of FimE. Error bars are the s.e.m. of quintuplicate measurements (totaln=240). Data symbol colours indicate the level of FimE induction shown ina. Grey line is the PLlacO-1 promoter (error bars are the s.e.m. of duplicate measurements). CV and mean in a strain with nativefimBandfimEare shown for comparison (HL1255). Black arrow indicates the direction of increasing FimB. Grey arrow indicates the direction of increasing IPTG for PLlacO-1::gfp. (c) CV as a function of mean expression with varying FimE and a fixed amount of FimB as indicated by the colour code ina. Error bars are the s.e.m. of quintuplicate measurements (totaln=240). Arrow indicates the direction of increasing FimE. Figure 7: The regulation of fimS by FimB and FimE. ( a ) A 6 × 8 ‘phase plane’ of representative histograms for the fimS system at different combinations of FimB and FimE expression. The phase space was measured in quintuplicate (HL4234). Panels from left to right show increasing FimE induction and panels from bottom to top show increasing FimB induction. Arrowheads highlight the small subpopulation of cells with the ON expression state. ( b ) The coefficient of variation (CV) as a function of mean expression with varying FimB and a fixed amount of FimE. Error bars are the s.e.m. of quintuplicate measurements (total n =240). Data symbol colours indicate the level of FimE induction shown in a . Grey line is the PLlacO-1 promoter (error bars are the s.e.m. of duplicate measurements). CV and mean in a strain with native fimB and fimE are shown for comparison (HL1255). Black arrow indicates the direction of increasing FimB. Grey arrow indicates the direction of increasing IPTG for PLlacO-1:: gfp . ( c ) CV as a function of mean expression with varying FimE and a fixed amount of FimB as indicated by the colour code in a . Error bars are the s.e.m. of quintuplicate measurements (total n =240). Arrow indicates the direction of increasing FimE. Full size image We calculated the CV from quintuplicate measurements at each combination of FimB and FimE induction and plotted the values as a function of the mean expression. These plots showed that increasing FimB at a fixed level of FimE produced loops as predicted ( Fig. 7b ). Furthermore, these loops shrink with increasing FimE as predicted. Another observation in agreement with the simulations is the ‘swirl’ pattern that occurs when FimE is increased at different fixed levels of FimB ( Figs 6c and 7c ). For comparison, we measured the CV and mean expression for an inducible promoter (PLlacO-1) and showed that it only produces a single CV for a given mean expression (grey line, Fig. 7b ). There are some differences between the experiments and the model. For example, the experimentally measured CV loops do not increase as much at high concentrations of FimB (that is, the last segment of the loop is not as steep) and the histograms show greater overlap between the OFF and ON expression states compared with the simulations ( Figs 6a,b and 7a,b ). This may be because the parameter values in the simulations were a priori estimates and may not be accurate for the: (i) transition rates among the promoter states (ON N , ON C and ON O ); and (ii) transcription initiation rate and the translation initiation rate. Altering these values makes the simulated histograms and CV loops more closely match the experiments ( Supplementary Fig. 9 ). Another difference between the experiments and simulations is leaky FimB and FimE expression (note: other studies also reported leaky FimB [26] and FimE [25] ). Leaky FimB expression accounts for the small numbers of cells that switch to the ON orientation at 0 μM IPTG (arrowheads, Fig. 7a ) and the higher starting point of the CV loops in the experiments. Leaky FimE expression explains why FimB is unable to switch most of the cells into the ON orientation at 0 nM aTc (in contrast to experiments without FimE; Figs 3 and 4 ) and it effectively eliminates the left two columns of the phase plane simulations ( Fig. 6a ). In summary, the experimental data are in relatively good agreement with the model and confirm its prediction that many different bimodal and unimodal distributions with different CV values can be produced with the same mean expression. There are differences between the experiments and the model, but this is not unexpected because the model was not designed to capture every detail of the system (for example, the model assumes a single copy of fimS rather than multiple copies as occurs in rapidly dividing cells [40] and it does not include extrinsic sources of gene expression noise [19] ); rather its purpose was to predict and provide an intuitive understanding of the basic properties of the system with the simplest assumptions and as few parameters as possible. This study describes a general strategy (FABMOS) for controlling the distribution of gene expression in a bacterial population and its successful implementation using a synthetic version of the fim system (FABMOS- fim ). One advantage of using the synthetic fim system for FABMOS is that it generates bimodality without feedback. Therefore, the expression levels of the states do not affect the frequency and bias of switching. Systems that generate bimodality through feedback can, under the right conditions, produce some behaviours that have been observed, such as a graded unimodal response [41] , [42] , [43] , [44] , [45] , [46] . However, the feedback makes it more difficult to tune phenotypic variation and mean expression. Bimodal distributions can also be generated by mechanisms that do not involve recombinases or feedback regulation, including DNA methylation [47] , sequestration [48] and futile cycles [49] , but how to tune the frequency and bias of switching with these mechanisms to implement FABMOS is unclear. Other advantages of the fim system include not requiring a specialized host or conditions [25] , that high FimB and FimE concentrations are not toxic and FimB regulates the frequency of both OFF-to-ON and ON-to-OFF transitions without affecting the bias. FABMOS could theoretically be constructed using alternative invertases and recombinases to FimB and FimE including Hin, Cre, Flp e , Bxb and phiC31 (refs 26 , 50 , 51 , 52 ). These alternative invertases and recombinases could be used in combination with the fim system to create FABMOS systems with more than two expression states. The FABMOS- fim system has potential applications in any area of experimental research and bioengineering where flexible control of phenotypic variation is desired. There are at least three broad areas of application. First, the FABMOS- fim system could be used as an experimental tool to study fundamental aspects of bacterial differentiation, ecology and evolution in which phenotypic variation is thought to have an important role but has not been fully investigated because of a lack of a system that allows phenotypic variation to be easily fine-tuned and varied independently of mean expression. Specifically, FABMOS could directly test theoretical models of how selection and phenotypic variation contribute to the fitness, robustness and evolvability of bacterial populations [4] , [53] , [54] , [55] , [56] . Testing these models will yield insights into processes that are important for human health and industrial applications, including bacterial pathogenesis, bacterial survival in response to antibiotics and stress, and cellular differentiation and cooperation in microbial communities [10] , [57] , [58] . Second, FABMOS- fim could increase adaptation and growth of bacterial populations in fluctuating environments. Specifically, it could generate two phenotypes that use different resources (for example, different carbon sources) and programme the frequency of switching between the phenotypes to be the same as the frequency of changes in the resources. This matching of the frequency of phenotypic switching and environmental fluctuations increases adaptation and thus strain fitness [4] , [5] , [8] . If the environment stops fluctuating, the same strain could be reprogrammed to have a unimodal distribution with every cell close to an optimal expression level to maximize growth and/or output of biosynthetic pathways [14] , [15] . Third, FABMOS- fim can create highly organized communities with distinct phenotypes to divide the effort of synthesizing ‘costly’ compounds [59] , [60] or separating incompatible biological processes (for example, nitrogen fixation and photosynthesis [13] ). Creating heterogeneous populations with cells performing different tasks can increase fitness and robustness [61] , result in more efficient use of resources [62] and enable cooperation that is essential for complex behaviours. Because of these benefits, some synthetic biologists have advocated engineering microbial strains that live in communities [59] , [61] as they commonly do in nature (note: the communities do not have to have different species for them to be beneficial [13] , [57] ). The FABMOS- fim system could create these different phenotypes and regulate their ratio, rates of switching and gene expression levels. Use of FABMOS in these second and third areas of application may help overcome the common problem that strains constructed in the lab often perform poorly in industrial settings [63] , [64] , [65] . In conclusion, frequency and bias modulation of switching is an experimentally validated strategy for the flexible and rational tuning of phenotypic variation and mean expression in bacterial populations. FABMOS could be harnessed to develop strains that are more adaptable, have faster growth rates, are more robust and are capable of generating communities with different phenotypes at specific ratios and levels of gene expression. Model and simulations To simulate the fim system, a transition rate matrix ( Q ) was created with values in the i th row and j th column ( q ij ) specifying the rate of transition from the i th state to the j th state of the promoter. Transitions from the ON O state to the ON N state, which occurred at a rate determined by the constant k M , generated an mRNA. Each mRNA was translated at a rate determined by the constant k P and degraded at a rate determined by the constant k −M . Each protein was degraded at a rate determined by the constant k −P . Therefore, the net rates of mRNA production, mRNA degradation, protein production and protein degradation in a cell are k M [ON O ], k −M [mRNA], k P [mRNA] and k −P [protein], respectively. All transition events including mRNA and protein production and degradation were stochastic and simulated using Gillespie’s algorithm [66] implemented in Matlab (R2008a and R2013b, Mathworks). Values for the rate constants are provided below. The first set of simulations ( Fig. 2 ; Supplementary Figs 1 and 2 ) were performed for 400 cells for a period representing 200 min, and each simulation was performed in duplicate. The initial fraction of the promoter in the ON orientation (ON N ) was determined by k 1 [FimB]/( k 1 [FimB]+ k −1 ([FimB]+[FimE])), except when [FimB]=0, in which case the initial fraction was 0.5. The initial mRNA and protein concentrations were zero. A small amount of random normally distributed background noise (mean of 1.0 arbitrary units (a.u.) and a s.d. of 0.5 a.u.) was added to the protein concentrations to account for autofluorescence (note: randomly generated negative values were set to zero). In Supplementary Fig. 1 , the model was altered so that: (i) transitions from ON to OFF occur at rate k −1 [FimE] (that is, FimB has no role in switching the orientation from ON to OFF); (ii) no transitions occur from ON C to OFF and ON O to OFF; or (iii) there are no transitions from ON N to ON C ( k 2 =0) and transcription occurs in the ON N state at a rate determined by k M . The rates of inversion from ON to OFF and OFF to ON were initially equal based on previous studies with k 1 = k −1 =0.0005 cells·min −1 (that is, 10 −2 inversion per generation assuming a generation time of 21 min). The rate constants for the conversion of the ‘naked’ promoter to the closed promoter complex ( k 2 ), the conversion of the closed promoter to the open promoter complex ( k 3 ) and the reverse transitions ( k −2 and k −3 , respectively) have not been determined in vivo . Therefore, we assigned arbitrary values of k 3 =100˙ k −3 = k 2 =100· k −2 =1 min −1 . k 2 and k 3 include the free concentrations of RNA polymerase and fimS sites, which are assumed to be constant. The mRNA degradation rate constant ( k −M ) was 0.1 min −1 based on an average mRNA half-life of 5 min (ln(2) per 5 min). Assuming an mRNA concentration of 10 mRNAs per cell [18] , the value for k M =1 mRNA·minute −1 . Fim proteins are stable and their clearance is primarily determined by the generation time, therefore the clearance rate constant k −P =0.03 min −1 (that is, ln(2) per 21 min). There are 100–500 type-1 fimbriae per cell [67] and each has 500–3,000 subunits of FimA and one each of FimD, FimF, FimG and FimH protein [29] . We selected a conservative value of 300 proteins·cell −1 , which equates to a translation rate constant k P =0.9 proteins˙(mRNA˙min) −1 (that is, a steady state mRNA concentration of 10 mRNAs·cell −1 multiplied by the translation rate constant of 0.9 proteins˙(mRNA˙min) −1 divided by the protein degradation rate of 0.03 min −1 yields 300 proteins·cell −1 ). Note: 1 protein·cell −1 ~1 nM. The second set of simulations ( Fig. 6 ) were performed as above, except that all simulations began in the OFF promoter state. Values for the rate constants are the same as for the first set, except that k −1 was reduced to 0.0001 cells·min −1 to reflect the observed bias. In addition, rate constants for transitions between the ON N , ON C and ON O promoter states were altered to k 3 = k −3 = k 2 = k −2 =1 min −1 . The normally distributed random noise that is added to the gene expression was modified to reflect the values of autofluorescence measured in a strain (MG1655) without the fluorescent reporter (that is, mean=0.60 a.u. and s.d.=0.66 a.u.). The output for the first and second set of simulations were very similar, which indicates the system is not fine-tuned to the values of k 3 , k −3 , k 2 and k −2 . Strains and plasmids Details of strains, plasmids and oligonucleotides are given in Supplementary Tables 1 and 2 . The strains and plasmids have been submitted to Addgene for distribution. The plasmid origin, T1 and t0 terminators and antibiotic resistance genes were obtained from the pZ system [16] . The gfp and lacIq genes were obtained from pGFPmut3.1 (Clontech) and pTrc99a (Pharmacia), respectively. The sources of the Asp terminator [68] and tetR [69] have been reported. fimB and fimE were generated by PCR amplification from MG1655 genomic DNA. The synthetic constitutive Pcon promoter was previously reported [68] and is derived from the sequence by Lanzer and Bujard [70] . Gene expression measurements Flow cytometry was performed using a Beckman-Coulter EPICS XL with an argon ion air-cooled laser and 525 nm band pass filter. The data were analysed using Flow Explorer 4.1 (R. Hoebe, University of Amsterdam, Netherlands) and software written in Matlab. The fraction of cells with ON expression was determined by counting the number of cells greater than a consistent saddle point in the histogram (12.0 fluorescence a.u.) and dividing the value by the total cell count. This method was more reproducible than fitting the distribution to two Gaussian (with logarithmic binning of GFP fluorescence) or two lognormal distributions, particularly when the fraction of one expression state was small. The typical protocol for measuring gene expression involved inoculating cells from overgrown cultures (1 in 4,500 dilution) into LB with 100 μg·ml −1 ampicillin and 34 μg·ml −1 chloramphenicol. The cells were grown for 2 h at 37 °C and 200 r.p.m. and then inoculated into fresh LB (1 μl in 3,000 μl dilution) with the appropriate concentrations of IPTG and aTc, and grown for another 240 min at 37 °C and 200 r.p.m. For experiments where we measured gene expression at multiple time points, the protocol was the same as above, except that after the first 2 h of growth we diluted 75 μl of inoculate into 3,000 μl of LB with the appropriate concentrations of antibiotic, IPTG and aTc and repeated this every 2 h to maintain a relatively constant cell density. Background autofluorescence measured in a strain without gfp (MG1655) had a mean of 0.60±0.01 a.u. and a s.d. of 0.66±0.01 a.u. Quantitative PCR Genomic DNA was extracted immediately after exponentially growing cells were collected using the Qiagen miniprep kit. Note: if cells were left on ice for ~1 h before DNA extraction, the fraction of ON orientation cells was 37.0±11.2% at 200 μM IPTG ( n =3) instead of the expected 75–85%. Two sets of PCR oligonucleotides were used to determine the relative fraction of OFF and ON orientation cells: one set amplified fimS in the OFF orientation (FimSInF and GFPseqR) and the other set amplified fimS in the ON orientation (FimSInF and FimEmidSeqF). Quantification of the products was performed by using IQSybR green supermix (Bio-Rad) and the iQ5 real-time PCR detection system (Bio-Rad). The fraction of cells with the fimS ON orientation was calculated by where and are the PCR efficiencies and CT OFF and CT ON are the threshold cycle (CT) values for the sets of oligonucleotides for the OFF and ON orientation, respectively. E OFF and E ON were 0.903±0.001 ( n =2) and 0.853±0.049 ( n =2), respectively, which was determined from the CT values obtained from a serial dilution (2 0 , 2 −1 , 2 −2 , 2 −3 and 2 −4 ) of PCR products with fimS in the OFF and ON orientations. The iQ5 software automatically assigned the CT values. How to cite this article: Hung, M. et al . Modulating the frequency and bias of stochastic switching to control phenotypic variation. Nat. Commun. 5:4574 doi: 10.1038/ncomms5574 (2014).